Generation of cellular immune memory and B-cell immunity is impaired by natural killer cells The goal of most vaccines is the induction of long-lived memory T and B cells capable of protecting the host from infection by cytotoxic mechanisms, cytokines and high-affinity antibodies. However, efforts to develop vaccines against major human pathogens such as HIV and HCV have not been successful, thereby highlighting the need for novel approaches to circumvent immunoregulatory mechanisms that limit the induction of protective immunity. Here, we show that mouse natural killer (NK) cells inhibit generation of long-lived virus-specific memory T- and B cells as well as virus-specific antibody production after acute infection. Mechanistically, NK cells suppressed CD4 T cells and follicular helper T cells (T FH ) in a perforin-dependent manner during the first few days of infection, resulting in a weaker germinal centre (GC) response and diminished immune memory. We anticipate that innovative strategies to relieve NK cell-mediated suppression of immunity should facilitate development of efficacious new vaccines targeting difficult-to-prevent infections. The development of vaccines has transformed global health by substantially reducing the threats associated with small pox, measles, polio and other infectious diseases. Nonetheless, infectious pathogens still contribute to a substantial proportion of worldwide mortality owing to the difficulty in developing vaccines against major infectious diseases such as HIV and hepatitis C virus (HCV). While the success of a vaccine depends, in large part, on their ability to mimic the induction of protective immunity that occurs after natural infection [1] , the correlates of immunity and basis for induction of such responses are markedly less apparent with pathogens (for example, HIV) that cause persistent infection. Moreover, the heightened mutability of HIV and HCV as well as the poor immunogenicity of conserved viral epitopes pose substantial barriers to vaccine-induced immunity [2] , [3] . Although the difficulties associated with these viruses as vaccine targets are inescapable, host immunoregulatory factors that limit the generation of protective immune responses may be amenable to interventions aimed at enhancing vaccine efficacy. An improved understanding of host factors that impair the induction of long-lived, protective antiviral immunity should permit the development of new vaccines that circumvent these immunoregulatory mechanisms to stimulate improved immune responses against challenging vaccine targets. Natural killer (NK) cells are innate immune effector lymphocytes that kill virus-infected cells and thereby represent an important component of antiviral immunity [4] . Recent evidence has highlighted the importance of another property of NK cells that of contributing to immune defense through regulation of adaptive immunity [5] . Target-cell killing and production of interferon gamma (IFN-γ) by NK cells has been reported to augment isotype class-switching by B cells [6] , [7] and to enhance the generation of memory T-cell responses [8] , [9] , [10] , [11] . In contrast, NK cells can inhibit adaptive antiviral immunity during persistent virus infection through production of immunosuppressive cytokines such as IL-10 (ref. 12 ), by modulating the function of antigen-presenting cells [13] , [14] , [15] , or by directly targeting T cells [16] , [17] , [18] . We recently demonstrated that NK cell-mediated lysis of activated CD4 T cells at an early stage of persistent infection of mice with the clone 13 strain of lymphocytic choriomeningitis virus (LCMV) was critical for prevention of fatal immunopathology [16] . This NK cell-mediated immunoregulation contributed to exhaustion of virus-specific T cells and viral persistence [16] , [18] , [19] . Here we explored the consequences of NK cell-mediated immune regulation on generation of memory T-cell responses and the induction of humoral immunity after acute infection of mice. Our results show that NK cells suppress the development of memory T-cell responses. In addition, we demonstrate that NK cells inhibit the development of B-cell responses resulting in fewer antigen-specific plasma cells and reduced levels of neutralizing antibodies. Together, these findings highlight the potential for NK cell-targeted treatments to improve immune responses in the context of vaccination or infection. Enhanced control of acute infection in absence of NK cells In the context of persistent LCMV [16] , [18] , [19] , NK cells have been shown to contribute to viral persistence by indirectly facilitating exhaustion and dysfunction of virus-specific CD8 T cells by lysing activated CD4 T cells [16] . Here we examined whether NK cells similarly had an impact on the control of virus replication during acute infection. Intraperitoneal (i.p.) inoculation of C57BL/6 mice with 5 × 10 4 plaque-forming units (p.f.u.) of the Armstrong or clone 13 strains of LCMV results in an acute infection cleared in ~1 week by virus-specific CD8 T cells. As previously shown [20] , NK cell deletion during the first 3 days of LCMV infection had little effect on LCMV titre. However, beginning on day 4 post infection, when the T-cell response begins to develop, viral titres were better controlled in the spleen during both acute Armstrong ( Fig. 1a ) and clone 13 ( Fig. 1b ) infections when NK cells were depleted (ΔNK) by i.p. administration of 25 μg of anti-NK1.1 monoclonal antibody (clone PK136) 1 day before infection. This dose of anti-NK1.1 selectively eliminates bona fide CD3 − /NK1.1 + NK cells while leaving NK/T cells intact [16] , [21] . Similarly, enhanced viral clearance was observed in NK cell-depleted mice during acute infection with 1.5 × 10 7 p.f.u. of Pichinde virus (PICV), a New World arenavirus ( Fig. 1c ). 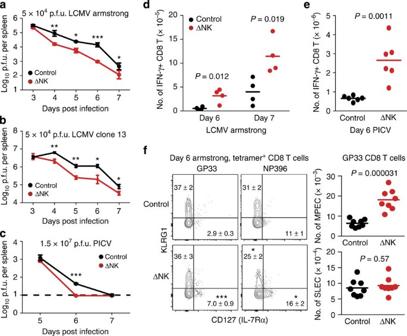Figure 1: NK cells limit T-cell-mediated antiviral immunity during acute infection. C57BL/6 mice (n=8 per group) were either treated i.p. with 25 μg NK cell-depleting anti-NK1.1 antibody (ΔNK) or a non-depleting isotype control (Control) 1 day before i.p. infection with (a,d,f) 5 × 104p.f.u. of LCMV Armstrong, (b) 5 × 104p.f.u. of LCMV clone 13 or (c,e) 1.5 × 107p.f.u. of PICV (n=3–4 per group). Statistical differences between groups were determined by Student’st-test and are denoted as *P<0.05, **P<0.01, ***P<0.001, or labelledPvalue. (a–c) Viral titres in the spleen (±s.e.m.) were determined at various time points p.i., where dotted line denotes limit of detection. (d,e) On days 6 or 7 after (d) LCMV Armstrong (n=4) or (e) day 6 of PICV infection (n=6), the quantities of IFN-γ-expressing (d) LCMV NP396-specific or (e) PICV NP38-specific CD44hiCD8 T cells were determined in the spleen by intracellular cytokine staining afterin vitrore-stimulation with virus-derived peptides. (f) On day 6 of LCMV Armstrong infection (n=8), virus-specific CD8 T cells were determined by staining with LCMV GP33- or NP396-loaded MHC class I tetramers. FACS plots display expression of KLRG1 and CD127 by gated CD8+CD44hitetramer-reactive CD8 T cells with the mean (±s.e.m.) proportion (in FACS plots) and number (graphs) of SLEC (KLRG1+CD127−) and MPEC (KLRG1−CD127+) phenotype cells among tetramer-reactive CD8 T cells. All data are representative of two to three independent experiments. Figure 1: NK cells limit T-cell-mediated antiviral immunity during acute infection. C57BL/6 mice ( n =8 per group) were either treated i.p. with 25 μg NK cell-depleting anti-NK1.1 antibody (ΔNK) or a non-depleting isotype control (Control) 1 day before i.p. infection with ( a , d , f ) 5 × 10 4 p.f.u. of LCMV Armstrong, ( b ) 5 × 10 4 p.f.u. of LCMV clone 13 or ( c , e ) 1.5 × 10 7 p.f.u. of PICV ( n =3–4 per group). Statistical differences between groups were determined by Student’s t- test and are denoted as * P <0.05, ** P <0.01, *** P <0.001, or labelled P value. ( a – c ) Viral titres in the spleen (±s.e.m.) were determined at various time points p.i., where dotted line denotes limit of detection. ( d , e ) On days 6 or 7 after ( d ) LCMV Armstrong ( n =4) or ( e ) day 6 of PICV infection ( n =6), the quantities of IFN-γ-expressing ( d ) LCMV NP396-specific or ( e ) PICV NP38-specific CD44 hi CD8 T cells were determined in the spleen by intracellular cytokine staining after in vitro re-stimulation with virus-derived peptides. ( f ) On day 6 of LCMV Armstrong infection ( n =8), virus-specific CD8 T cells were determined by staining with LCMV GP33- or NP396-loaded MHC class I tetramers. FACS plots display expression of KLRG1 and CD127 by gated CD8 + CD44 hi tetramer-reactive CD8 T cells with the mean (±s.e.m.) proportion (in FACS plots) and number (graphs) of SLEC (KLRG1 + CD127 − ) and MPEC (KLRG1 − CD127 + ) phenotype cells among tetramer-reactive CD8 T cells. All data are representative of two to three independent experiments. Full size image Since altered viral clearance could have an impact on antigen presentation, we examined the proportion and number of various antigen-presenting cells in the spleens at different times after infection with the Armstrong or clone 13 strains of LCMV ( Supplementary Fig. 1 ). There were few differences between control and ΔNK mice during either infection with regards to the proportion of CD8α + CD11c + dendritic cells (DC), PDCA-1 + B220 + plasmacytoid DCs or F4/80 + CD11b + macrophages (Mφ) among lineage-negative (CD3 − CD19 − NK1.1 − ) cells. However, there were small increases in the number of CD8α + and CD11b + DCs on days 4 and 5 after LCMV clone 13 infection, and in the number of plasmacytoid DC on day 5 of Armstrong or day 3 of clone 13 infection. Likewise, there were similar levels of the cytokines IFN-γ, tumour necrosis factor (TNF), interleukin-10 (IL-10), IL-6 and IL-2 in the sera of control and ΔNK mice during infection with LCMV Armstrong or clone 13 ( Supplementary Fig. 2 ). Together, this suggests that inflammation and antigen-presenting cell frequencies are relatively similar in the presence and absence of NK cells, despite altered levels of replicating virus. Depressed antiviral T-cell responses in presence of NK cells Control of acute infections with LCMV and PICV is mediated by virus-specific CD8 T cells, and increased numbers of LCMV- ( Fig. 1d ) and PICV-specific ( Fig. 1e ) IFN-γ-expressing CD8 T cells were in the spleens of NK cell-depleted mice relative to NK cell-replete controls on days 6 and 7 of infection, coincident with the diminished virus burden in the absence of NK cells ( Fig. 1a,c ). The phenotype of responding CD8 T cells during acute infection can be a faithful indicator of the propensity of these cells to contract or become memory cells. Specifically, memory precursor effector cells (MPECs) express high levels of the IL-7 receptor alpha chain (IL-7Rα or CD127) and low levels of killer cell lectin-like receptor subfamily G member 1 (KLRG1), whereas short-lived effector cells (SLECs) display the inverse (CD127 − KLRG1 + ) phenotype [22] . Here LCMV GP33- and NP396-specific CD8 T cells were identified in the spleen on day 6 of LCMV Armstrong infection by peptide-loaded major histocompatibility complex (MHC) class I tetramer staining, and then examined for expression levels of KLRG1 and CD127. The proportion and number of MPEC (CD127 + KLRG1 − ) virus-specific CD8 T cells was increased among GP33 ( Fig. 1f ) and NP396 (Control=2.3±0.38 × 10 4 MPEC; ΔNK=9.6±2.0 × 10 4 MPEC, n =8, 2 replicates, P =0.000028, Student’s t -test) tetramer-reactive CD8 T cells in the absence of NK cells. Whereas the number and percentage of the SLEC phenotype (CD127 − KLRG1 + ) GP33-tetramer-reactive CD8 T cells was not changed by NK cell depletion ( Fig. 1f ), there was a reduced proportion ( Fig. 1f ) but increased number (Control=6.4±0.57 × 10 4 SLEC; ΔNK=17.0±5.0 × 10 4 MPEC, n =8, two replicates, P =0.018, Student’s t -test) of NP396-tetramer-reactive CD8 T cells with a SLEC phenotype that likely reflects the increased total number of NP396-specific CD8 T cells ( Fig. 1d ) in the absence of NK cells. Similar results were obtained during acute infection with the clone 13 strain of LCMV ( Supplementary Fig. 3a ). Thus, NK cells repress the number of virus-specific CD8 T cells and the generation of MPECs during acute virus infection. NK cells restrict the generation of memory T cells An increase in the magnitude of primary T-cell responses during acute infection in the absence of NK cells, as well as the increased frequency of MPEC phenotype cells, could contribute to an enhanced generation of memory T cells after infection of NK cell-depleted mice. In fact, depletion of NK cells before an acute course of infection with the clone 13 strain of LCMV resulted in enhanced numbers of memory CD8 ( Fig. 2a ) and CD4 ( Fig. 2b ) T cells 7 weeks later. Moreover, the proportion of memory NP396-specific CD8 ( Fig. 2c ) and GP61-specific CD4 T cells ( Fig. 2d ) capable of simultaneous production of multiple cytokines (left: IFN-γ/TNF; right: IFN-γ/TNF/IL-2) was increased in mice that had been depleted of NK cells during acute infection. Similar results were observed at 12 weeks after acute infection with the clone 13 strain of LCMV ( Supplementary Fig. 3b ). The magnitudes of LCMV-specific CD4 ( Fig. 2e ) and CD8 ( Supplementary Fig. 3c ) memory T-cell responses were also enhanced by NK cell depletion during acute infection with the Armstrong strain of LCMV. Likewise, ablation of NK cells during acute LCMV Armstrong infection boosted the proportion of LCMV-specific memory CD8 and CD4 T cells capable of simultaneous production of multiple cytokines ( Fig. 2f ). In a similar manner, depletion of NK cells before acute PICV infection resulted in an enhanced proportion ( Fig. 3a ) and number ( Fig. 3b ) of virus-specific memory CD8 T cells 73 days later. Notably, subdominant responses against the PICV-encoded epitopes NP205 and NP122 (ref. 23 ) were markedly enriched. Thus, NK cells can regulate the magnitude, breadth and the quality of the memory T-cell response. 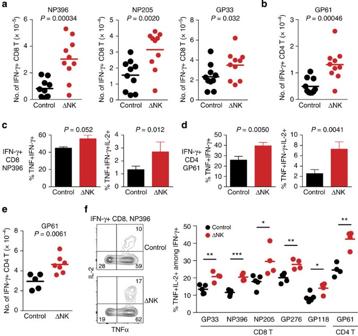Figure 2: Magnitude and quality of antiviral memory T-cell responses are impaired by NK cells. C57BL/6 mice (n=9–10 per group) were either treated i.p. with 25 μg anti-NK1.1 antibody (ΔNK) or isotype control (Control) 1 day before i.p. infection with 5 × 104p.f.u. of (a–d) LCMV clone 13 or (e,f) LCMV Armstrong. (a,b) The numbers of splenic IFN-γ+LCMV-specific (a) CD8 and (b) CD4 T cells were determined 49–52 d.p.i. by intracellular cytokine staining afterin vitrore-stimulation with virus-derived peptides. The fraction of IFN-γ+LCMV (c) NP396-specific CD8 and (d) GP61-specific CD4 T cells (±s.e.m.) co-expressing TNF-α (left) or TNF-α and IL-2 (right) is graphed (n=10 per group). (e) The number of IFN-γ+GP61-specific CD4 T cells was determined in the spleen 36 days after infection with LCMV Armstrong. (f) The fraction of IFN-γ+CD8 and CD4 T cells co-expressing TNF-α and IL-2 on day 202 of LCMV Armstrong infection is graphed for mice (n=4–5 per group) treated with isotype (Control) or anti-NK1.1 antibody (ΔNK) 1 day before infection. Significant differences between groups were determined by Student’st-test and are displayed as *P<0.05, **P<0.01, ***P<0.001 or actualPvalue. Data ina–dare pooled from two independent experiments, whilee,fare representative of two similar experiments. Figure 2: Magnitude and quality of antiviral memory T-cell responses are impaired by NK cells. C57BL/6 mice ( n =9–10 per group) were either treated i.p. with 25 μg anti-NK1.1 antibody (ΔNK) or isotype control (Control) 1 day before i.p. infection with 5 × 10 4 p.f.u. of ( a – d ) LCMV clone 13 or ( e , f ) LCMV Armstrong. ( a , b ) The numbers of splenic IFN-γ + LCMV-specific ( a ) CD8 and ( b ) CD4 T cells were determined 49–52 d.p.i. by intracellular cytokine staining after in vitro re-stimulation with virus-derived peptides. The fraction of IFN-γ + LCMV ( c ) NP396-specific CD8 and ( d ) GP61-specific CD4 T cells (±s.e.m.) co-expressing TNF-α (left) or TNF-α and IL-2 (right) is graphed ( n =10 per group). ( e ) The number of IFN-γ + GP61-specific CD4 T cells was determined in the spleen 36 days after infection with LCMV Armstrong. ( f ) The fraction of IFN-γ + CD8 and CD4 T cells co-expressing TNF-α and IL-2 on day 202 of LCMV Armstrong infection is graphed for mice ( n =4–5 per group) treated with isotype (Control) or anti-NK1.1 antibody (ΔNK) 1 day before infection. Significant differences between groups were determined by Student’s t -test and are displayed as * P <0.05, ** P <0.01, *** P <0.001 or actual P value. Data in a – d are pooled from two independent experiments, while e , f are representative of two similar experiments. 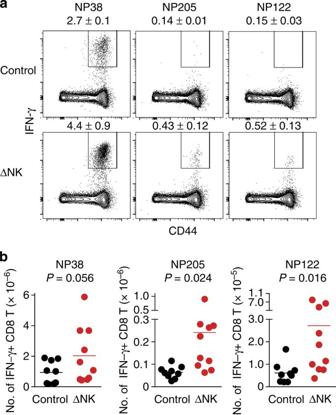Figure 3: Greater magnitude and breadth of memory CD8 T-cell responses when primed in absence of NK cells. Following selective depletion of NK cells (ΔNK) or treatment with control antibody (Control), C57BL/6 mice were infected with 1.5 × 107p.f.u. of PICV i.p. On day 73 p.i., the (a) proportion (mean±s.e.m.,n=5 per group) and (b) number (n=9–10 per group) of IFN-γ-expressing PICV-specific CD8 T cells were determined in the spleen by intracellular cytokine staining afterin vitrore-stimulation with virus-derived peptides. Data inaare representative of two independent experiments, while data from two experiments are pooled inb. Statistical differences between groups were determined by Student’st-test. Full size image Figure 3: Greater magnitude and breadth of memory CD8 T-cell responses when primed in absence of NK cells. Following selective depletion of NK cells (ΔNK) or treatment with control antibody (Control), C57BL/6 mice were infected with 1.5 × 10 7 p.f.u. of PICV i.p. On day 73 p.i., the ( a ) proportion (mean±s.e.m., n =5 per group) and ( b ) number ( n =9–10 per group) of IFN-γ-expressing PICV-specific CD8 T cells were determined in the spleen by intracellular cytokine staining after in vitro re-stimulation with virus-derived peptides. Data in a are representative of two independent experiments, while data from two experiments are pooled in b . Statistical differences between groups were determined by Student’s t -test. Full size image A previous study found that NK cells restricted the number of ovalbumin (OVA)-specific OT-I TCR-transgenic memory CD8 T cells generated after immunization with OVA in lipopolysaccharide and reported that the NK cell receptor, NKG2D, played an important role in this regulation [24] . However, we had previously demonstrated that NKG2D, which is encoded by the gene klrk1 , was not required for virus-induced NK cell-mediated lysis of CD4 T cells [16] . Likewise, NKG2D was dispensable in the regulation of virus-specific memory T cells described in our current study. The frequency of PICV NP38 tetramer-reactive memory CD8 T cells was comparable in wild-type and NKG2D-deficient mice 54 days after acute PICV infection ( Supplementary Fig. 4a ). NK cell depletion augmented memory responses to a similar extent regardless of whether NKG2D was present. Similarly, NK cells repressed the frequency of IFN-γ + LCMV NP396-specific memory CD8 T cells 49 days after acute infection with 5 × 10 4 p.f.u. of LCMV clone 13 irrespective of the expression of NKG2D ( Supplementary Fig. 4b ). Thus, NK cell-mediated suppression of virus-specific memory T-cell responses is a general feature of different virus infections and occurs independently of NKG2D. NK cells impair T FH cell responses On the basis of our previous demonstration that virus infection triggers NK cell lysis of activated CD4 T cells [16] , we hypothesized that NK cells would suppress the development of follicular helper CD4 T cells (T FH ) [25] and subsequent humoral immune responses. In fact, NK cell-depleted mice harboured a greater proportion of both activated (CD44 hi CD49d + ) and T FH (CXCR5 + PD-1 + ) cells among gated CD4 + T cells compared with control mice on day 6 of LCMV Armstrong infection ( Fig. 4a , left three panels). Notably, the percentage of gated activated (CD44 hi CD49d + ) CD4 T cells with a T FH phenotype (CXCR5 + PD-1 + ) was also enhanced in NK cell-depleted mice ( Fig. 4a , far right panel). Thus, the augmented quantity of activated CD4 T cells in the absence of NK cells comprises increased numbers of both T FH (CXCR5 + PD-1 + ) and non-T FH (CXCR5 − PD-1 − ) cells ( Fig. 4b ). 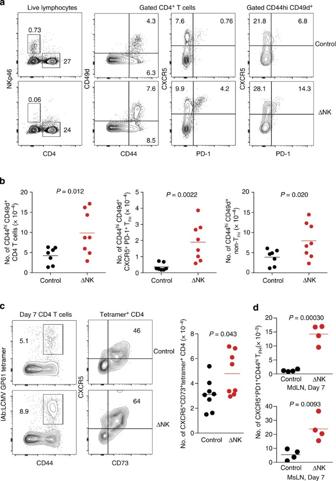Figure 4: NK cells suppress TFHresponses during infection. Groups of C57BL/6 mice were infected with 5 × 104p.f.u. (i.p.) of (a–c) LCMV Armstrong (n=7–8 per group) or (d) 3 × 105c.f.u. (i.p.) ofL. monocytogenes(n=4 per group) 1 day after treatment with anti-NK1.1 (ΔNK) or isotype control (Control). (a,b) On day 6 p.i., live singlet lymphocytes in the inguinal LN (left panel,a) were determined to be NK cells (NKp46+CD4−) or CD4 T cells (NKp46−CD4+). Gated CD4 T cells (middle panels,b) were analysed for activation markers CD44 and CD49d or TFHmarkers PD-1 and CXCR5. Activated (CD44hiCD49d+) CD4 T cells (right panel,a) were further analysed for expression of PD-1 and CXCR5. Representative FACS plots and proportions are shown in (a), while total numbers of activated (left panel,b: CD44hiCD49d+), TFH(middle panel, b: CD44hiCD49d+CXCR5+PD-1+) and non-TFH(right panel,b: CD44hiCD49d+CXCR5−PD-1−) splenic CD4 T cells for individual mice are shown inb. (c) On day 7 of infection, splenic CD4 T cells (left panel) were stained with anti-CD44 and LCMV GP61-loaded MHC class II tetramers to determine LCMV-specific CD4 T cells. These cells were examined for markers of TFHphenotype CD73 and CXCR5 (middle panel). The total number of LCMV GP61-specific TFHcells (CD73+CXCR5+CD44hiTetramer+) in eight individual mice per group is plotted the in right panel. (d) Number of TFH(CD44hiCD49d+CXCR5+PD-1+) in the mediastinal (MdLN) and mesenteric (MsLN) LNs on day 7 ofL. monocytogenesinfection. Data are pooled from two independent experiments, and statistically significant differences were determined by Student’st-test. Figure 4: NK cells suppress T FH responses during infection. Groups of C57BL/6 mice were infected with 5 × 10 4 p.f.u. (i.p.) of ( a – c ) LCMV Armstrong ( n =7–8 per group) or ( d ) 3 × 10 5 c.f.u. (i.p.) of L. monocytogenes ( n =4 per group) 1 day after treatment with anti-NK1.1 (ΔNK) or isotype control (Control). ( a , b ) On day 6 p.i., live singlet lymphocytes in the inguinal LN (left panel, a ) were determined to be NK cells (NKp46 + CD4 − ) or CD4 T cells (NKp46 − CD4 + ). Gated CD4 T cells (middle panels, b ) were analysed for activation markers CD44 and CD49d or T FH markers PD-1 and CXCR5. Activated (CD44 hi CD49d + ) CD4 T cells (right panel, a ) were further analysed for expression of PD-1 and CXCR5. Representative FACS plots and proportions are shown in ( a ), while total numbers of activated (left panel, b : CD44 hi CD49d + ), T FH (middle panel, b: CD44 hi CD49d + CXCR5 + PD-1 + ) and non-T FH (right panel, b : CD44 hi CD49d + CXCR5 − PD-1 − ) splenic CD4 T cells for individual mice are shown in b . ( c ) On day 7 of infection, splenic CD4 T cells (left panel) were stained with anti-CD44 and LCMV GP61-loaded MHC class II tetramers to determine LCMV-specific CD4 T cells. These cells were examined for markers of T FH phenotype CD73 and CXCR5 (middle panel). The total number of LCMV GP61-specific T FH cells (CD73 + CXCR5 + CD44 hi Tetramer + ) in eight individual mice per group is plotted the in right panel. ( d ) Number of T FH (CD44 hi CD49d + CXCR5 + PD-1 + ) in the mediastinal (MdLN) and mesenteric (MsLN) LNs on day 7 of L. monocytogenes infection. Data are pooled from two independent experiments, and statistically significant differences were determined by Student’s t -test. Full size image Increased proportions of LCMV GP61-specific CD4 T cells were also evident in the spleens of NK cell-depleted mice on day 7 of LCMV Armstrong infection, as determined with MHC class II tetramer staining ( Fig. 4c , left). Remarkably, the proportion ( Fig. 4c , middle) and number ( Fig. 4c , right) of these LCMV-specific CD4 T cells displaying a T FH phenotype, here determined by expression of CXCR5 and CD73 (ref. 26 ), was measurably increased in the absence of NK cells. This suggests that the increased T FH response in NK cell-depleted mice is not merely a consequence of enhanced T-cell activation, but that these T FH cells are preferentially expanded as part of a larger augmentation of the virus-specific CD4 T-cell response. Expression of inducible T-cell costimulator (ICOS), which is critical for T FH functionality [27] , [28] , was similar as determined by the mean fluorescence intensity (MFI) of staining (Control, 1,145±176 ICOS MFI (±denotes s.e.m. throughout the text); ΔNK 1,296±58 ICOS MFI; n =4, one of two replicates, P =0.15, Student’s t -test) on tetramer-reactive CD4 T cells with a T FH phenotype (CXCR5 + CD73 + ) in control and NK cell-depleted mice. Enhanced numbers of T FH cells were also apparent in the spleen 6 days after PICV (Control=9.2±2.9 × 10 4 T FH cells; ΔAGM1=13.6±0.53 × 10 4 T FH cells, n =4, one of two replicates, P =0.050, Student’s t -test) or 7 days after Listeria monocytogenes infection ( Fig. 4d ), suggesting that NK cell inhibition of T FH is a general feature of diverse systemic infections. NK cell suppression of GC responses NK cell killing of activated CD4 T cells [16] and suppression of T FH responses would likely have profound consequences for CD4 T-cell-dependent aspects of humoral immunity, including the formation of germinal centres (GCs). Consistent with this hypothesis, T FH and GC B-cell (GL7 + Fas + CD19 + B220 + ) responses were concomitantly enhanced in the spleen and lymph nodes (LNs) on days 6–7 of LCMV Armstrong (5 × 10 4 p.f.u.) infection ( Fig. 5a ). We also observed an increased proportion and number of GC B cells in NK cell-depleted mice 14 days after infection with LCMV Armstrong ( Fig. 5b ), a time when the GC response is at its peak. Enumeration of the number of peanut agglutinin (PNA)- and anti-B220-reactive GC areas in longitudinal sections of the spleen on day 14 of infection revealed that control and NK cell-depleted spleens appeared to harbour a similar number of these PNA + B220 + structures ( Fig. 5c ), suggesting that NK cells may restrict the cellularity of GCs more so than their frequency during acute infection. 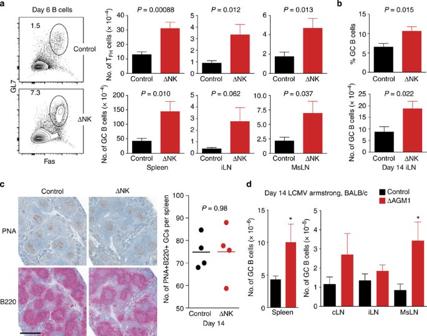Figure 5: NK cells suppress germinal center responses after acute virus infection. (a–c) C57BL/6 mice were depleted of NK cells with anti-NK1.1 or administered an equivalent amount of isotype control antibody (Control) 1 day before infection with 5 × 104p.f.u. LCMV Armstrong i.p. (a) Six to 7 d.p.i., the proportions and numbers of GC (Fas+GL7+) B cells (B220+CD19+) and TFHcells (±s.e.m.) were determined in the spleen (n=12 per group), inguinal (iLN;n=12–16 per group) and mesenteric (MsLN;n=12–16 per group) nodes. (b) The fraction and number of TFHcells in the iLN on day 14 of infection (n=8 per group). (c) PNA and anti-B220 staining of GC reactions in formalin-fixed spleen sections on day 14 of infection (scale bar, 500 μ). PNA+B22O+GC areas were enumerated in a complete spleen section from four mice per group. (d) The frequency of GC B cells in the spleen and LNs on day 14 of LCMV Armstrong (5 × 104p.f.u. i.p.) infection in groups of BALB/c mice (n=8 per group) that received normal rabbit serum (control) or 20 μl anti-asialoGM1 (ΔAGM1) one day before infection. All results are representative of two similar experiments. Significant differences between control and NK cell-depleted groups are displayed as *P<0.05 or givenPvalue, as determined by Student’st-test. Figure 5: NK cells suppress germinal center responses after acute virus infection. ( a – c ) C57BL/6 mice were depleted of NK cells with anti-NK1.1 or administered an equivalent amount of isotype control antibody (Control) 1 day before infection with 5 × 10 4 p.f.u. LCMV Armstrong i.p. ( a ) Six to 7 d.p.i., the proportions and numbers of GC (Fas + GL7 + ) B cells (B220 + CD19 + ) and T FH cells (±s.e.m.) were determined in the spleen ( n =12 per group), inguinal (iLN; n =12–16 per group) and mesenteric (MsLN; n =12–16 per group) nodes. ( b ) The fraction and number of T FH cells in the iLN on day 14 of infection ( n =8 per group). ( c ) PNA and anti-B220 staining of GC reactions in formalin-fixed spleen sections on day 14 of infection (scale bar, 500 μ). PNA + B22O + GC areas were enumerated in a complete spleen section from four mice per group. ( d ) The frequency of GC B cells in the spleen and LNs on day 14 of LCMV Armstrong (5 × 10 4 p.f.u. i.p.) infection in groups of BALB/c mice ( n =8 per group) that received normal rabbit serum (control) or 20 μl anti-asialoGM1 (ΔAGM1) one day before infection. All results are representative of two similar experiments. Significant differences between control and NK cell-depleted groups are displayed as * P <0.05 or given P value, as determined by Student’s t -test. Full size image Anti-NK1.1 administration could affect other NK1.1-expressing cells, including NK/T cells. However, our regimen of 25 μg of anti-NK1.1 did not deplete NK/T cells [16] and NK cell depletion enhanced both T FH ( Supplementary Fig. 5a ) and GC B-cell numbers ( Supplementary Fig. 5b ) on day 8 of Armstrong infection in the LNs of CD1d-deficient ( Cd1d −/− ) mice, which are devoid of classical invariant NK/T cells. Moreover, depletion of NK cells in BALB/c mice using a limiting dose of anti-asialo GM1 antibody (ΔAGM1) that eliminates most NK cells while leaving T-cell responses intact [29] also enhanced the resulting number of T FH cells in the spleen on day 8 after infection with 5 × 10 4 p.f.u. LCMV Armstrong i.p. (Control=5.5±1.5 × 10 5 T FH cells; ΔAGM1=16.2±3.0 × 10 5 T FH cells, n =3, one of two replicates, P =0.033, Mann–Whitney test) and caused an appreciable increase in the number of GC B cells after LCMV Armstrong infection of BALB/c ( Fig. 5d ) and C57BL/6 (data not shown) mice. Increased GC B-cell responses were also observed in the spleen 6 days after infection (Control=9.4±3.3 × 10 4 GC B cells, ΔNK1.1=19.6±8.7 × 10 4 GC B cells, n =8, total of two replicates, P =0.016, Student’s t -test) with a low dose of LCMV clone 13 (5 × 10 4 p.f.u. i.p.) and on day 8 after infection (Control=5.1±0.96 × 10 5 GC B cells, ΔNK1.1=10.3±1.2 × 10 5 GC B cells, n =8, total of two replicates, P =0.0023, Student’s t -test) with a high intravenous (i.v.) dose of the LCMV clone 13 (2 × 10 6 p.f.u.). Finally, a fraction of the observed GC B-cell response could have been a response against bovine serum present in our viral stocks. Thus, we utilized high-titre LCMV Armstrong preparations diluted 400-fold in serum-free Hank’s balanced salt solution (inguinal lymph node (iLN) 14 days post infection (d.p.i. ), Control=5.5±0.59% GC among B cells, ΔNK1.1=9.6±0.75% GC among B cells, n =23, four replicates, P =0.00005, Student’s t -test) to demonstrate that this phenomenon is independent of bovine serum contamination. Together, these results demonstrate that NK cell suppression of GC reactions is a feature of different types of infections and is not a nuance of C57BL/6 mice or the anti-NK1.1 antibody used to selectively deplete NK cells. NK cells limit antibody and long-lived humoral immunity The GC response primarily functions to facilitate the differentiation of B cells into long-lived plasma cells that populate the bone marrow as well as to enable somatic hypermutation of immunoglobulin sequences [30] . When infected with LCMV Armstrong in the absence of NK cells, C57BL/6 mice harboured a modestly increased number of LCMV-specific antibody-secreting cells (ASCs) in the spleen 3 weeks after infection, as determined by ELISPOT against LCMV-infected and mock-infected baby hamster kidney (BHK) lysates ( Fig. 6a ). Importantly, while LCMV-specific ASCs were largely absent from the bone marrow of NK cell-sufficient mice at this early time point 21 d.p.i., there was already a substantial number of these cells present in the bone marrow of NK cell-depleted mice ( Fig. 6a ). Moreover, the number of long-lived bone marrow ASC, which likely represent plasma cells, was enhanced in mice inoculated with virus in the absence of NK cells relative to NK cell-sufficient control mice 74–82 days after infection ( Fig. 6b ). Thus, NK cell suppression of GC responses is associated with reduced frequencies of LCMV-specific ASCs for months after infection. 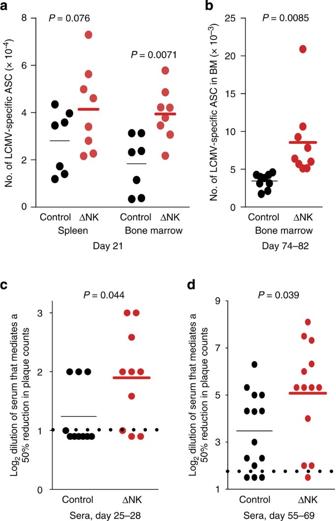Figure 6: Enhanced LCMV-specific antibody responses in absence of NK cells. C57BL/6 mice (n=7–9 per group) were depleted of NK cells (ΔNK) or treated with isotype antibody (control) 1 day before i.p. infection with 5 × 104p.f.u. LCMV Armstrong. Spleen and bone marrow cells were collected and subjected to the ELISPOT analysis of ASC frequencies: (a) 21 or (b) 74–82 d.p.i. (c) Sera from mice (n=10 per group) on day 28 p.i. was analysed for the ability to neutralize LCMV in a plaque reduction assay, which is graphed as log2of the greatest dilution that could mediate a ≥50% reduction in p.f.u. (d) Neutralizing antibody titres were also determined as incfor sera from mice (n=13–14 per group) 55–69 days after LCMV Armstrong infection. Dotted lines represent limit of detection. Data are pooled from two to three independent experiments, and statistical significance of differences determined by Student’st-test. Figure 6: Enhanced LCMV-specific antibody responses in absence of NK cells. C57BL/6 mice ( n =7–9 per group) were depleted of NK cells (ΔNK) or treated with isotype antibody (control) 1 day before i.p. infection with 5 × 10 4 p.f.u. LCMV Armstrong. Spleen and bone marrow cells were collected and subjected to the ELISPOT analysis of ASC frequencies: ( a ) 21 or ( b ) 74–82 d.p.i. ( c ) Sera from mice ( n =10 per group) on day 28 p.i. was analysed for the ability to neutralize LCMV in a plaque reduction assay, which is graphed as log 2 of the greatest dilution that could mediate a ≥50% reduction in p.f.u. ( d ) Neutralizing antibody titres were also determined as in c for sera from mice ( n =13–14 per group) 55–69 days after LCMV Armstrong infection. Dotted lines represent limit of detection. Data are pooled from two to three independent experiments, and statistical significance of differences determined by Student’s t -test. Full size image Somatic hypermutation of immunoglobulin sequences in the GC facilitates affinity maturation and development of high-affinity neutralizing antibodies (nAbs) [30] . Such nAbs usually appear very late (that is, 3 months) after LCMV infection [31] , [32] and are relatively weak in comparison with responses after infections with other viruses, including vesicular stomatitis virus [33] . Serum from C57BL/6 mice 4 weeks after infection with LCMV Armstrong demonstrated little ability to neutralize LCMV ( Fig. 6c ) in a plaque reduction assay [34] , wherein most sera were completely devoid of such activity. A greater proportion of sera from NK cell-depleted Armstrong-infected mice demonstrated a measureable level of neutralizing activity, and, although the levels were very low compared with viruses that potently induce nAbs (for example, vesicular stomatitis virus) [33] , the mean neutralizing activity was slightly elevated in NK cell-depleted mice ( Fig. 6c ). The levels of LCMV-specific nAb ( Fig. 6d ) were also increased in the sera of NK cell-depleted mice relative to control mice at later time points after acute LCMV Armstrong infection. However, there were wide variations in antibody responses within experiments as well as between stocks of virus. Thus, despite a substantial enhancing effect of NK cell depletion on T FH and GC B-cell responses, statistically significant reductions in virus-specific antibody responses in the presence of NK cells were modest and somewhat variable between experiments. B-cell-independent suppression of T FH by NK cells Examination of very early time points (day 5 p.i.) of LCMV infection revealed that NK cell depletion resulted in an enhanced number of T FH (CXCR5 + PD-1 + ) cells ( Fig. 7a ) before the measureable detection of GC responses at levels that exceed those observed in uninfected mice ( Fig. 7b ). GC B-cell responses were not detectable until day 6 or 7 p.i. in the spleen and other LNs ( Fig. 5a ). Thus, NK cell-mediated suppression of T FH responses can be measured at times preceding appearance of GC B-cell responses. 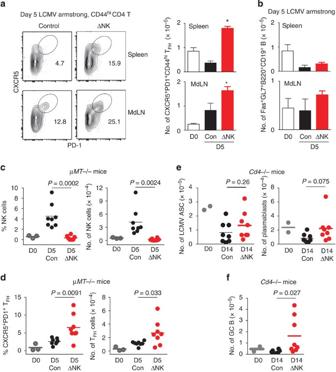Figure 7: Inhibition of humoral immunity by NK cells involves CD4 T cells. C57BL/6 mice were depleted of NK cells (ΔNK) or treated with isotype antibody (Control, Con) 1 day before i.p. infection with 5 × 104p.f.u. of LCMV Armstrong. Significant differences between control and NK cell-depleted groups were determined by Student’st-test and are displayed as *P<0.05 or actualPvalue. On day 5 after Armstrong infection, frequencies of (a) TFH(CXCR5+PD-1+CD44hiCD4+) cells and (b) GC (Fas+GL7+B220+CD19+) B cells (±s.e.m.) were determined (n=4 per group) in the spleen and MdLN. Results are representative of two similar experiments. (c,d)μMT−/− mice (n=3 for naive;n=8 per group for infected) were depleted of NK cells (ΔNK) or treated with control antibody (Con) 1 day before infection with 5 × 104p.f.u. (i.p.) LCMV Armstrong, or were left uninfected (D0). The proportion (left) and number (right) of (c) NKp46+CD3−NK cells or (d) CD44hiCXCR5+PD-1+CD4 T cells was determined in the spleen on day 5 of infection. (e,f)Cd4−/− mice were depleted of NK cells (ΔNK) or were treated with control antibody (Con) 1 day before infection with 5 × 104p.f.u. (i.p.) LCMV Armstrong (n=2 for naive;n=8 per group for infected). (e) The numbers of plasmablast cells (CD138+IgD−CD19+B220+), LCMV-specific antibody-secreting cells and (f) GC (Fas+IgD−CD19+B220+) B cells were determined in the spleen on day 14 of infection. All results are pooled from two independent experiments. Figure 7: Inhibition of humoral immunity by NK cells involves CD4 T cells. C57BL/6 mice were depleted of NK cells (ΔNK) or treated with isotype antibody (Control, Con) 1 day before i.p. infection with 5 × 10 4 p.f.u. of LCMV Armstrong. Significant differences between control and NK cell-depleted groups were determined by Student’s t -test and are displayed as * P <0.05 or actual P value. On day 5 after Armstrong infection, frequencies of ( a ) T FH (CXCR5 + PD-1 + CD44 hi CD4 + ) cells and ( b ) GC (Fas + GL7 + B220 + CD19 + ) B cells (±s.e.m.) were determined ( n =4 per group) in the spleen and MdLN. Results are representative of two similar experiments. ( c , d ) μMT −/− mice ( n =3 for naive; n =8 per group for infected) were depleted of NK cells (ΔNK) or treated with control antibody (Con) 1 day before infection with 5 × 10 4 p.f.u. (i.p.) LCMV Armstrong, or were left uninfected (D0). The proportion (left) and number (right) of ( c ) NKp46 + CD3 − NK cells or ( d ) CD44 hi CXCR5 + PD-1 + CD4 T cells was determined in the spleen on day 5 of infection. ( e , f ) Cd4 −/− mice were depleted of NK cells (ΔNK) or were treated with control antibody (Con) 1 day before infection with 5 × 10 4 p.f.u. (i.p.) LCMV Armstrong ( n =2 for naive; n =8 per group for infected). ( e ) The numbers of plasmablast cells (CD138 + IgD − CD19 + B220 + ), LCMV-specific antibody-secreting cells and ( f ) GC (Fas + IgD − CD19 + B220 + ) B cells were determined in the spleen on day 14 of infection. All results are pooled from two independent experiments. Full size image To determine whether B cells played a part in NK cell inhibition of T FH responses, we infected B-cell-deficient ( μMT −/− ) [35] mice with LCMV Armstrong. On day 5 p.i., the percentage and number of NK cells in the spleen was increased in infected control mice relative to their naive and NK cell-depleted counterparts ( Fig. 7c ). Of greater significance, the proportion and number of T FH cells was elevated in the spleen at 5 d.p.i. in NK cell-depleted mice relative to nondepleted controls ( Fig. 7d ). Thus, NK cells are capable of impairing T FH responses in the absence of an intact B-cell compartment. Role for CD4 T cells in augmented humoral immunity To examine the role of CD4 T cells in the NK cell control of the GC B-cell response, we depleted CD4 T-cell-deficient cd4 −/− mice [36] of NK cells before infection with LCMV. As expected for a T-cell-dependent humoral response, LCMV-specific ASC and plasmablast (CD138 + IgD − ) B cells were largely undetectable or below levels present in uninfected mice in the spleens of cd4 −/− mice on day 14 of infection, regardless of the presence or absence of NK cells ( Fig. 7e ). Surprisingly, a weak GC B-cell response was measurable in NK cell-depleted cd4 −/− mice but not in NK cell-replete cd4 −/− controls ( Fig. 7f ). Moreover, the number of IgD − -activated B cells was increased in the absence of NK cells in cd4 −/− mice (Control=2.5±1.7 × 10 5 IgD − B cells, ΔNK1.1=5.0±2.2 × 10 5 IgD − B cells, n =8, two replicates, P =0.023, Student’s t -test). Overall, the weak B-cell responses and marginal changes in these responses upon NK cell depletion in CD4 T-cell-deficient mice suggests that NK cell suppression of CD4 T-cell responses likely plays a more prominent role in the inhibition of humoral immune responses than any direct effects of NK cells upon B cells. NK cells act during initial days of acute infection To determine at what stage of infection NK cell suppression of memory T-cell and B-cell immune responses takes place, we first examined the duration of NK cell depletion during infection. To our surprise, a single injection of anti-NK1.1 antibody 1 day before LCMV Armstrong infection maintained an effective depletion of more than 50% of circulating NK cells for 4 weeks ( Fig. 8a ). Therefore, an alternative strategy was needed to evaluate the timing of the NK cell-suppressive effect. Towards this end, anti-NK1.1 antibody was administered 3 or 6 days after infection. Two weeks after infection, virus-specific IFN-γ-expressing T-cell ( Fig. 8b ) and GC B-cell ( Fig. 8c ) responses were enhanced in the spleen and LNs, respectively, of mice depleted of NK cells before infection (day −1) but not in mice depleted of NK cells on days 3 or 6 after infection. These results suggest that NK cells suppress T- and B-cell responses at a very early stage of infection (before day 3), consistent with the prior studies by our group [16] and others [19] in the persistent LCMV clone 13 infection model. 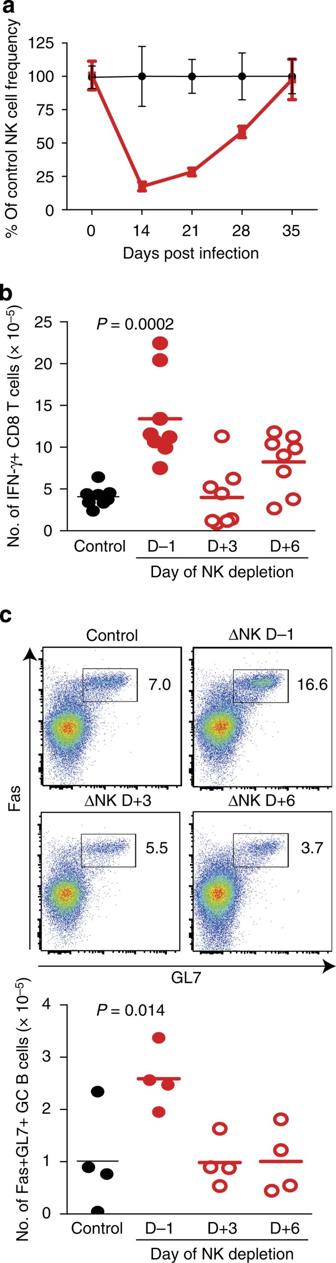Figure 8: NK cell suppression of humoral and cellular immunity occurs at an early stage of infection. Before infection (D −1) with 5 × 104p.f.u. (i.p.) of the Armstrong strain of LCMV, C57BL/6 mice (n=4 per group) were treated with 25 μg of anti-NK1.1 (ΔNK) or isotype (control) antibody. (a) The frequencies of NK cells (±s.e.m.) were determined in peripheral blood at various times post infection, and are plotted as a fraction of nondepleted control mice at each time point. (b,c) Additional groups of mice were administered a single dose of anti-NK1.1-depleting antibody at later time points (day 3 (D+3) or day 6 (D+6) p.i.). (b) LCMV-specific CD8 T-cell responses in the spleen (n=8 per group) were measured by intracellular cytokine staining on day 14 p.i. afterin vitrore-stimulation with virus-derived peptides. (c) Numbers of GC B cells (n=4 per group) were determined in the iLN on day 14 p.i. Results are pooled from two independent experiments, and statistically significant differences were determined by Student’st-test. Figure 8: NK cell suppression of humoral and cellular immunity occurs at an early stage of infection. Before infection (D −1) with 5 × 10 4 p.f.u. (i.p.) of the Armstrong strain of LCMV, C57BL/6 mice ( n =4 per group) were treated with 25 μg of anti-NK1.1 (ΔNK) or isotype (control) antibody. ( a ) The frequencies of NK cells (±s.e.m.) were determined in peripheral blood at various times post infection, and are plotted as a fraction of nondepleted control mice at each time point. ( b , c ) Additional groups of mice were administered a single dose of anti-NK1.1-depleting antibody at later time points (day 3 (D+3) or day 6 (D+6) p.i.). ( b ) LCMV-specific CD8 T-cell responses in the spleen ( n =8 per group) were measured by intracellular cytokine staining on day 14 p.i. after in vitro re-stimulation with virus-derived peptides. ( c ) Numbers of GC B cells ( n =4 per group) were determined in the iLN on day 14 p.i. Results are pooled from two independent experiments, and statistically significant differences were determined by Student’s t -test. Full size image Role for perforin in NK cell suppression of humoral immunity Cytotoxicity is a major effector function exerted by NK cells in the elimination of virus-infected and transformed target cells. To determine whether cytotoxicity is involved in NK cell regulation of humoral immunity, perforin-deficient mice ( prf1 −/− ) [37] were depleted of NK cells or treated with isotype control antibody 1 day before infection with LCMV Armstrong. At an early stage of infection before the severe pathology associated with lack of viral control and aberrant responses of prf1 −/− CD8 T cells, the proportion ( Fig. 9a ) and number ( Fig. 9b ) of T FH cells was measurably enhanced by NK cell depletion in wild-type mice. T FH cells were also elevated in prf1 −/− mice regardless of the presence or absence of NK cells. NK cell depletion resulted in enhancement of splenic T FH responses in wild-type mice and in lpr mice with a dysfunctional Fas/FasL axis [38] ( Fig. 9c ). Therefore, NK cell suppression of humoral immunity is independent of Fas/FasL but requires a perforin-mediated pathway. In support of a role for perforin in NK cell-mediated suppression of the GC response, a marked increase in the spontaneous degranulation of NK cells as determined by ex vivo CD107a/b staining [39] was observed in the spleen and LNs following infection with LCMV ( Fig. 9d ). While the nature of the NK cell cytotoxicity receptors potentially involved in this NK cell-mediated immunoregulation are unclear, we did observe that NKG2D was similarly dispensable for NK cell-mediated suppression of T FH and GC B cells ( Supplementary Fig. 4c ) and virus-specific T-cell memory responses after acute infection ( Supplementary Fig. 4a,b ). 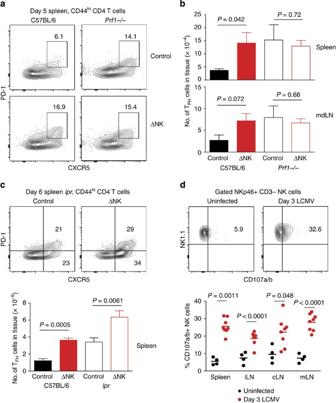Figure 9: NK cell suppression of TFHresponses depends on perforin. (a–c) Groups of C57BL/6,prf1−/− orlprmice (n=8 per group) were depleted of NK cells (ΔNK) or administered control antibody (Control) 1 day before infection with LCMV Armstrong (5 × 104p.f.u.). (a) Representative staining of TFHmarkers CXCR5 and PD-1 on activated (CD44hi) CD4 T cells in the spleen 5 d.p.i. (b) Numbers of TFHcells (PD-1+CXCR5+CD44hiCD4+) in the spleen and melon on day 5 p.i. (±s.e.m.). (c) Proportion and number of TFHcells (±s.e.m.) in the spleen on day 6 of infection of C57BL/6 andlprmice. (d)Ex vivodegranulation measured by CD107a/b staining of NKp46+CD3−NK cells in the spleen and LNs of uninfected or LCMV-infected (day 3 p.i.), and total number of degranulating (CD107a/b+) NK cells (n=8 per group) is plotted. Results are pooled from two independent replicate experiments, and statistically significant differences were determined using Student’st-test. Figure 9: NK cell suppression of T FH responses depends on perforin. ( a – c ) Groups of C57BL/6, prf1 −/− or lpr mice ( n =8 per group) were depleted of NK cells (ΔNK) or administered control antibody (Control) 1 day before infection with LCMV Armstrong (5 × 10 4 p.f.u.). ( a ) Representative staining of T FH markers CXCR5 and PD-1 on activated (CD44hi) CD4 T cells in the spleen 5 d.p.i. ( b ) Numbers of T FH cells (PD-1 + CXCR5 + CD44 hi CD4 + ) in the spleen and melon on day 5 p.i. (±s.e.m.). ( c ) Proportion and number of T FH cells (±s.e.m.) in the spleen on day 6 of infection of C57BL/6 and lpr mice. ( d ) Ex vivo degranulation measured by CD107a/b staining of NKp46 + CD3 − NK cells in the spleen and LNs of uninfected or LCMV-infected (day 3 p.i. ), and total number of degranulating (CD107a/b + ) NK cells ( n =8 per group) is plotted. Results are pooled from two independent replicate experiments, and statistically significant differences were determined using Student’s t -test. Full size image These results demonstrate that NK cells inhibit the induction of humoral immunity and memory T cells following an array of acute infections. Notably, NK cells contributed to delayed and diminished GC reactions that were subsequently associated with decreased LCMV-specific antibody and plasma cell responses. Moreover, the quantity and quality of T-cell memory was reduced by NK cell activities during acute infection. Consideration of these suppressive functions of NK cells in the context of vaccination could unveil innovative means of enhancing humoral and cellular responses against vaccine-associated antigens. The enhancement of LCMV-specific ASC and antibody responses in mice that had been transiently depleted of NK cells during acute infection represents a compelling new way to think about the contribution of innate responses to the development of protective humoral immunity. Increased generation of bone marrow plasma cells (that is, ASCs) and improved elaboration of nAbs in the absence of NK cells indicates that there are measureable consequences of NK cell suppression of the GC response, including restriction of somatic hypermutation and affinity maturation of virus-specific antibody [30] . Yet, despite the profound effects of NK cell depletion on T FH and GC B-cell responses, differences in neutralizing antibody formation were modest in most experiments and sometimes not statistically significant. An explanation may be that the curtailed antigen levels after NK cell depletion of acutely infected mice, likely resulting from the enhanced CD8 T-cell responses ( Fig. 1 ), are insufficient to efficiently promote the expansion of the B-cell response and affinity maturation of antibodies. The consistent twofold increase in the number of bone marrow ASCs coupled with the more marginal and sporadic gains in nAb titres could reflect the delicate balance between the need for B cells in the GC to undergo repeated rounds of somatic hypermutation versus the propensity of these cells to undergo terminal differentiation into long-lived plasma cells [30] , which no longer mutate their antigen receptor. In future studies, it will be of great interest to examine the molecular changes in these GC B cells in the presence and absence of NK cells in order to evaluate expression of Blimp1/Prdm1 (ref. 40 ), which determines plasma cell differentiation, as well as to examine the extent of somatic hypermutation of immunoglobulin sequences in these cells. Moreover, it will be important to determine whether NK cells influence the development of vaccine-induced nAbs against clinically relevant pathogens, such as HIV. Examination of the underlying factors contributing to enhanced humoral immune responses in the absence of NK cells showed that in the absence of CD4 T cells, plasmablasts and LCMV-specific ASC were largely absent in the spleen of LCMV-infected mice and that the accelerated appearance of differentiated T FH cells in NK cell-deficient mice preceded the development of GC B-cell responses. These findings suggest that the suppressive effect of NK cells on B-cell responses is a consequence of NK cell-mediated inhibition of T FH responses. In fact, we confirmed that B cells are not required for CD4 T cells to differentiate into T FH cells, and that NK cell-mediated suppression of T FH responses occurs even in the absence of B cells. Nevertheless, plasmablast responses were trending higher in NK cell-depleted cd4 −/− mice, while activated IgD low and GC B-cell responses were enhanced by NK cell depletion in the absence of CD4 T cells. This could reflect an additional effect of NK cells, beyond the suppression of T FH responses, that is either mediated directly upon B cells or via regulation of other leukocytes (that is, NK/T cells, basophils or CD8 T cells) [41] , [42] , [43] capable of providing B-cell help. Following LCMV infection, NK cells in the spleen and LNs displayed increased levels of the degranulation markers CD107a and CD107b compared with uninfected mice, suggesting that NK cells within these tissues of infected mice are cytotoxic. The loss of granule-mediated cytotoxicity in perforin-deficient mice resulted in an increased number of T FH cells after LCMV infection that was similar to levels observed in NK cell-depleted perforin-sufficient wild-type mice. Moreover, NK cell depletion failed to further enhance the T FH response in perforin-deficient mice. In contrast, Fas-deficient lpr mice were readily amenable to NK cell-depletion-mediated enhancement of T FH responses, suggesting that the Fas/FasL system is dispensable in this NK cell-mediated suppression. These results are consistent with our previous finding that NK cells can lyse CD4 T cells [16] , and point to a prominent role for perforin-mediated cytolysis in NK cell suppression of humoral immunity. Nevertheless, we have not ruled out a direct perforin-dependent effect of NK cells on B cells. B cells, however, may be protected from the direct cytolytic effects of NK cells because B cells express high levels of CD48 (ref. 44 ), which delivers negative signals to murine NK cells [45] . It remains unclear whether the NK cell-mediated control of T FH cells is because of a direct effect of NK cells upon differentiated T FH cells or a result of a diminished number of activated CD4 T cells capable of differentiating into T FH cells. There was an increased proportion of activated CD4 T cells with a T FH phenotype, suggesting that these cells are preferentially inhibited. However, there were increased numbers of both T FH and non-T FH CD4 T cells in NK cell-depleted mice, indicating that the suppression exerted by NK cells may be more broadly applied to multiple lineages of differentiated CD4 T cells. Notably, the suppressive activity of NK cells upon both T- and B-cell responses was primarily mediated during the initial 3 days of infection, which may indicate that NK cells interfere with an early step in the activation and differentiation of CD4 T cells. Future studies will also aid in determining whether NK cells influence T-cell activation and T FH differentiation via direct effects on CD4 T cells, as we previously described in a chronic infection model [16] , or through the inhibition of antigen-presenting cell function [13] , [19] , [46] , [47] . The simplest explanation for increased numbers of memory T cells lies in the substantially elevated magnitude of primary T-cell responses during acute infection. If a constant fraction of cells is lost during contraction, this larger pool of effector T cells should directly translate to a greater quantity of memory T cells. However, memory cell differentiation is not a stochastic process, but has instead been linked to the expression of the IL-2 (CD25) and IL-7 (CD127) receptor alpha chains on activated T cells with enhanced potential to develop into long-lived memory cells [48] , [49] . As early as 2 or 3 d.p.i., precursors of memory T cells can be distinguished on the basis of low expression of the IL-2 receptor alpha chain [48] , [50] . Notably, this early fate determination of virus-specific T cells coincides with the peak of NK cell-mediated suppression of virus-specific T cells observed during the first 3 days of LCMV clone 13 infection [16] , [19] . Therefore, diminished antiviral memory T-cell responses after infection in the presence of NK cells may be a consequence of NK cell-mediated elimination of precursors of these memory T cells at very early stages of the response. In fact, analysis of tetramer-reactive LCMV-specific CD8 T cells at an early stage of infection demonstrated that NK cells are associated with a reduced fraction and number of T cells with a memory precursor (CD127 + KLRG1 − ) phenotype. Thus, NK cells may restrict memory T-cell development by limiting the differentiation of memory precursor cells. It is important to note that NK cells can also exert beneficial effects on T- and B-cell responses during vaccination. Notably, NK cell-derived IFN-γ can promote antigen-presenting cell functionality, T H 1 differentiation of T cells, and isotype class-switching in B cells. Moreover, immunization of mice with apoptotic splenocytes expressing membrane-bound OVA resulted in development of memory OVA-specific CD8 T-cell responses that were enhanced by the presence of NK cells during priming [8] . In contrast, immunization of mice with OVA protein admixed with bacterial lipopolysaccharide resulted in impaired generation of OVA-specific memory CD8 T cell as a consequence of NK cell-mediated suppression [24] . We speculate that inflammation associated with virus infection triggers NK cell-mediated suppression of memory T-cell development, such that the occurrence of this inhibition may vary widely depending on the nature of the vaccine regimen (that is, live virus versus protein subunit) or the adjuvant (that is, alum versus CpG DNA) used. Therefore, careful selection of adjuvants to optimize the beneficial effects of inflammation on memory T-cell development while minimizing interference by NK cells represents one viable approach to enhance vaccine efficacy. In addition, further studies aimed at determining whether NK cells similarly suppress memory T and B cells will reveal whether NK cell-mediated immunoregulation can have compound effects upon prime-boost vaccination strategies or during re-vaccination of immune individuals. Mice C57BL/6, BALB/c, cd4 −/− , μMT −/− , prf1 −/− and lpr mice were purchased from The Jackson Laboratories (Bar Harbor, ME). Klrk1 −/− (ref. 51 ) on a C57BL/6 background were obtained from Bojan Polic (University of Rijeka). C57BL/6 cd1d −/− were obtained from Mark Exley [52] (University of Manchester) or David Hildeman [53] (CCHMC), respectively. Male mice at 6–12 weeks of age (at onset of infection) were routinely utilized in experiments. Mice were housed under pathogen-free conditions, and experiments were performed using the ethical guidelines approved by the Institutional Animal Use and Care Committees of the University of Massachusetts Medical School and Cincinnati Children’s Hospital Medical Center. In many experiments, randomization was achieved by randomly assigning mice within a cage to different experimental groups or by modulating the processing order of the mice at the time of harvest. In vivo NK cell depletion One day before infection, selective depletion [16] of NK cells was attained through a single i.p. injection of 25 μg per mouse anti-NK1.1 monoclonal antibody (PK136) or 25 μg per mouse of a control mouse IgG2a (C1.18.4) produced by Bio-X-Cell (West Lebanon, NH). Alternatively, NK Cells were depleted through a single i.p. injection with 20 μl of anti-asialo GM1 (Wako Biochemicals, Richmond, VA) diluted in 180 μl of Hank’s balanced salt solution (HBSS) or 20 μl of normal rabbit serum (Wako Pure Chemical Industries, Japan) diluted in 180 μl HBSS. Infections The Armstrong and clone 13 strains of LCMV were propagated in BHK21 cells [54] . Virus was titrated by plaque assay on Vero cells from American Type Culture Collection (ATCC, Manassas, VA). Mice were inoculated with 5 × 10 4 p.f.u. of LCMV Armstrong i.p. The clone 13 strain of LCMV was administered at a dose of 5 × 10 4 i.p. or 2 × 10 6 p.f.u. i.v. PICV was prepared in BHK21 cells and titrated by plaque assay on Vero cells [55] . PICV was administered i.p. at a dose of 1.5 × 10 7 p.f.u. per mouse. L. monocytogenes (strain 10403S) was grown in the brain heart infusion (BHI) medium at 37 °C to early log-phase (OD 600 0.1), washed, suspended in PBS and inoculated i.v. at a dose of 3 × 10 5 colony-forming units [56] . Peptides and tetramers Synthetic peptides (90% purity by reverse phase-HPLC) representing LCMV-encoded epitopes recognized by T cells in the context of MHC were purchased from 21st Century Biochemicals. These peptides include the IA b -presented LCMV GP61-80 or GP64-80 epitope (GLKGPDIYKGVYQFKSVEFD); D b -presented LCMV GP33-41 (KAVYNFATC), LCMV GP276-286 (SGVENPGGYCL), LCMV NP396-404 (FQPQNGQFI) and PICV NP122-132 (VYEGNLTNTQL), and the K b -presented LCMV NP205-212 (YTVKYPNL), LCMV GP118-125 (ISHNFCNL), PICV NP205-212 (YTVKFPNM) and PICV NP38-45 (SALDFHKV). Production of PICV NP38-45-loaded MHC class I tetramers was previously described [57] . LCMV GP33-41 (KAVYNFATC) and NP396 (FQPQNGQFI)-loaded H-2D b tetramers were produced at the NIH Tetramer Facility. Class I tetramer staining was performed at room temperature for 45 min before addition of surface antibodies. LCMV GP61-80 epitope-loaded Ia b tetramers were acquired from David Hildeman (CCHMC), and class II tetramer staining was performed at 37 °C for 75 min before surface-staining with fluorescent antibodies. Antibodies and FACS analysis Fluorescently labelled antibodies purchased from BD Biosciences (San Diego, CA) include the following: CD95/Fas (Jo2, 1:200), GL7 (1:200), CD44 (IM7, 1:200), CD4 (RM4-5, 1:400), IL-2 (JES6-5H4, 1:100), NK1.1 (PK136, 1:200), CD45R/B220 (RA3-6B2, 1:200) and CD3ε (500A2, 1:300). Antibodies purchased from eBioscience (San Diego, CA) include the following: GL7 (1:200) and PD-1 (RMPI-30, 1:200). Antibodies purchased from BioLegend (San Diego, CA) include the following: CD8α (53-6.7, 1:200), CD8β (53-5.8, 1:400), IgD (11-26c.2a, 1:200), CD19 (6D5, 1:200), NK1.1 (PK136, 1:200), NKp46 (29A1.4, 1:50), TNFα (MP6-XT22, 1:200), CXCR5 (L138D7, 1:50), CD45R/B220 (RA3-6B2, 1:200), FR4 (12A5, 1:200), CD73 (TY/11.8, 1:200), F4/80 (BM8, 1:200), CD49d (R1-2, 1:200), ICOS (C398.4A, 1:200), CD11b (M1/70, 1:200), CD138 (281-2, 1:200), CD127 (A7R34, 1:200), KLRG1 (2F1/KLRG1, 1:200), CD107a (1D4B, 1:200), CD107b (M3/84, 1:200) and CD4 (GK1.5, 1:400). Antibodies purchased from Tonbo Biosciences include the following: CD44 (IM7, 1:200), IFNγ (XMG1.2, 1:1,000), CD3ε (145-2C11, 1:300), CD19 (1D3, 1:200), B220 (RA3-6B2, 1:200), CD11c (N418, 1:200) and CD16/32 (2.4G2, 1:200). Antibodies purchased from Miltenyi Biotec include the following: CD49b/DX5 (DX5, 1:200) and CD8α (53-6.7, 1:200). Cells were collected on a LSR II or LSR Fortessa cytometer equipped with the FACSDiva software (BD Biosciences), and data were analysed with the FlowJo software (Tree Star, Ashland, OR). Lymphocyte preparation and intracellular cytokine assay Single-cell leukocyte suspensions were prepared from spleens and LNs by mechanical homogenization of tissues between glass slides. Single-cell suspensions from various tissues were plated at 2 × 10 6 cells per well in 96-well plates and either immediately subjected to flow staining or first stimulated for 5 h at 37 °C with 1 μM viral peptide in the presence of brefeldin A and 0.2 U ml −1 recombinant human IL-2. Cells were then incubated with a 1:200 dilution of anti-CD16/32 (Fc block 2.4G2) in flow cytometry buffer (HBSS+5% fetal calf serum) and stained for 20 min at 4 °C with various combinations of fluorescently tagged antibodies. Alternatively, cells were first stained at 4 °C with tetramers for 40 min before the 20-min surface stain. Following staining, cells were washed and permeabilized with BD Cytofix/Cytoperm solution and then stained in BD Perm/Wash using antibodies specific for various intracellular cytokines. ASC assay Multiscreen HA filter ELISPOT plates (EMD Millipore) were coated with 100 μl of LCMV-Armstrong-infected BHK cell lysates or mock-infected BHK cell lysates at 4° overnight. Plates were UV-irradiated for 10 min and the supernatant was aspirated. Plates were washed once with PBS containing 0.1% Tween-20 (PBST) and twice with PBS, and then blocked with 100 μl of media for 3 h at room temperature. While plates were blocking, bone marrow cells and splenocytes from infected mice were harvested and serially diluted threefold in serum-free RPMI-1640 media. After 3 h, media were aspirated from the plate and 100 μl of bone marrow or spleen cells were added to each well and incubated with antigen for 4–5 h at 37 °C. After incubation, the plate was washed three times with PBS and three times with PBST. A 100-μl volume of PBST with 1% FBS and a 1:1,000 dilution of biotin anti-mouse IgG (Life Technologies) was added to each well and incubated overnight at 4 °C. The plate was washed four times with PBST before the addition of 100 μl of PBST with 1% FBS and a 1:1,000 dilution of streptavidin-horseradish peroxidase (Life Technologies) to each well. The plate was incubated at room temperature for 1 h, washed three times with PBST and three times with PBS, and then 100 μl of AEC substrate (Life Technologies) was added to each well. The plate was incubated at room temperature for 5 min and wells were washed with tap water. Plate was air-dried and spots were counted manually with a dissecting microscope. PNA staining of GC reactions Tissues from mice were placed into 10% buffered formalin. Slides were prepared and stained in the CCHMC Pathology Core. GCs were enumerated by immunohistochemistry using anti-B220 antibody (1:50, BD Biosciences) and anti-PNA (Vector Labs 1:50). All imaging was performed using an Aperio digital slide scanner at × 20 magnification, and images were analysed using the ImageScope software (Leica Biosystems). Luminex analysis of cytokine expression IFN-γ, TNFα, IL-2, IL-6, IL-10 and IL-21 cytokine concentrations in serum supernatants were determined in the Cincinnati Children’s Hospital Medical Center Research Flow Cytometry Core by Alyssa Sproles using enzyme-linked immunosorbent assay using Milliplex Multiplex kits (Millipore, Billerica, MA) according to the manufacturer’s protocol. Briefly, in a 96-well black plate, 25 μl of sample in duplicate was incubated with 25 μl antibody-coated beads overnight at 4 °C on a plate shaker. Plates were then washed twice on a vacuum apparatus, and 25 μl of secondary antibody was added and incubated at room temperature for 1 h while shaking. Finally, 25 μl of streptavidin-R-phycoerythrin was added directly to the secondary antibody and incubated for 30 min at room temperature with shaking. Plates were then washed twice and 100 μl of sheath fluid was added. Plates were shaken for 5 min and then read using luminex technology on the Bio-Plex (Bio-Rad, Hercules, CA). Concentrations were calculated from standard curves using recombinant proteins. Degranulation assay Single-cell suspensions were kept warm and quickly prepared from spleen and LNs of uninfected C57BL/6 mice or from mice 3 days after infection with LCMV. Cells were plated at 2 × 10 6 cells per well in 96-well plates and were stimulated for 4 h at 37 °C with brefeldin A (0.2 μl ml −1 ) and a 1:200 dilution of fluorescein isothiocyanate-conjugated CD107a (1D4B) and CD107b (M3/84) for a total volume of 200 μl per well. Following incubation, cells were washed and stained for various other surface markers. Plaque reduction (nAb) assay Neutralizing activity of LCMV-specific antibodies present in sera was measured using a plaque reduction assay [34] . Briefly, heat-inactivated serum was subjected to serial twofold dilutions. Then, 100 μl of diluted serum was incubated with 100 μl of defined quantities of LCMV Armstrong for 1.5 h at 37 °C. The amount of infectious virus remaining was measured by the standard plaque assay on Vero cells. Results are reported as the log 2 of the greatest dilution able to mediate a 50% reduction in plaque counts. Statistical analysis Experimental results are consistently presented as mean±s.e.m. Statistical differences between control and NK cell-depleted groups were determined using a Mann–Whitney test or the two-tailed unpaired Student’s t -test depending on whether data demonstrated Gaussian distribution and equal variance. With both tests, a P value of <0.05 was considered significant. Graphing and statistical analyses were performed using either Microsoft Excel or GraphPad Prism (San Diego, CA). In occasional instances, researchers performing the analysis were blinded to the experimental groupings of the animals or serum samples. We estimated the sample size considering the variation and the mean of the distribution. How to cite this article: Rydyznski, C. et al. Generation of cellular immune memory and B-cell immunity are impaired by natural killer cells. Nat. Commun. 6:6375 doi: 10.1038/ncomms7375 (2015).